Effective localized collection and identification of airborne species through electrodynamic precipitation and SERS-based detection Various nanostructured sensor designs currently aim to achieve or claim single molecular detection by a reduction of the active sensor size. However, a reduction of the sensor size has the negative effect of reducing the capture probability considering the diffusion-based analyte transport commonly used. Here we introduce and apply a localized programmable electrodynamic precipitation concept as an alternative to diffusion. The process provides higher collection rates of airborne species and detection at lower concentration. As an example, we compare an identical nanostructured surfaced-enhanced Raman spectroscopy sensor with and without localized delivery and find that the sensitivity and detection time is improved by at least two orders of magnitudes. Localized collection in an active-matrix array-like fashion is also tested, yielding hybrid molecular arrays on a single chip over a broad range of molecular weights, including small benzenethiol (110.18 Da) and 4-fluorobenzenethiol (128.17 Da), or large macromolecules such as anti-mouse IgG (~150 kDa). Detection of chemical agents in the gas phase has attracted much attention because of the applications and potential for explosives detection and environmental monitoring [1] , [2] , [3] , [4] . The detection of small molecules and airborne species at low concentration commonly requires sensing schemes where the analytes are absorbed on a surface. The process of absorption and precipitation is, therefore, critical to the detection limit of the analytes. This is true for all the established gas-phase sensing concepts including gas chromatography [5] , ion mobility spectrometry [6] , [7] , mass spectrometry [8] , metal-semiconductor-metal-based sensors [1] , [9] , [10] , chemical field effect transistors [11] , nanocantilever [12] , infrared detection [13] and surfaced-enhanced Raman spectroscopy (SERS) [14] , [15] . Interestingly, most of the more recently reported sensing schemes aim at increasing the sensitivity to a single molecular level [16] and use diffusion as a mechanism for transport that leads to a collection efficiency of the airborne species, which is not optimized. Schedin et al. [16] as an example, reported the detection of a single molecule from a carrier gas at a concentration of 1 p.p.m. The experiments used a micrometer-sized graphene sensor. The authors concluded that ‘Large arrays of such sensors would increase the catchment area [17] , allowing higher sensitivity for short-time exposures and the detection of active (toxic) gases in as minute concentrations as practically desirable.’ In other words, it becomes increasingly difficult to detect and capture molecules on the basis of diffusion in cases where the active sensing area is reduced unless the question of localized delivery is addressed. Effective collection on a small sensing area is not possible based on diffusion alone and the employment of a directed force will be required to solve the problem of transport. Both the thermophoretic and Coulomb force can be utilized to transport the analytes from a distance away to the sensing surface. At practical temperature gradients the thermophoretic force, however, remains low compared with concepts that use electrostatic precipitation [4] . Different from prior methods [5] , [6] , [7] , [8] , [9] , [10] , [11] , [12] , [13] , [14] , [15] , this article reports and applies a programmable localized electrodynamic precipitation concept to collect, spot and detect airborne species in an active-matrix array like fashion. The approach discussed here does not use mechanical masks [18] , [19] or high-precision contact-printing robots [20] , [21] to deliver the analytes to desired points and provides programmability with a lateral resolution that is several orders of magnitudes higher. Molecules of one type are directed from a space that is centimeters away to specific sensing regions and areas with 100 nm control over the lateral position and spot size. The detection scheme is demonstrated using a SERS-sensitized nanostructured surface. It employs the standardized ‘Ag film over Nanosphere (AgFON) substrate’ [14] , [22] , and compares the results with and without programmable localized electrodynamic precipitation and finds that SERS signals are enhanced by a factor of 615 compared with identical sensor surfaces. The process is able to detect charged benzenethiol (BT) molecules at an estimated level of 1.5 p.p.b. (parts per billion) within 10 s, as a comparison, to detect uncharged molecules using a standard mechanism of diffusion a concentration of 6 p.p.m. (parts per million) is required. The reported process is applied to produce hybrid molecular arrays on a single chip over a broad range of molecular weights including small molecules such as BT (110.18 Da) and 4-fluorobenzenethiol (4-FBT) (128.17 Da) or large macromolecules such as anti-mouse IgG proteins (~150 kDa). 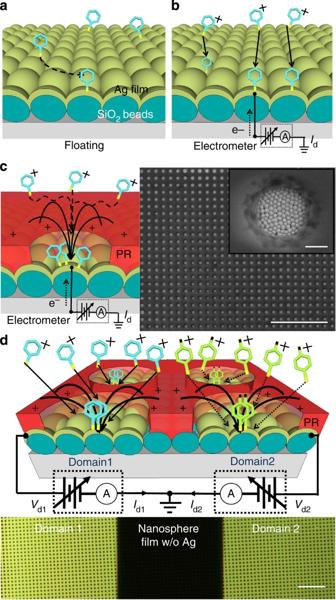Figure 1: Advanced localized collection and spotting of airborne species for gas sensor applications. (a,b) A nanostructured substrate commonly used in SERS called AgFON, which uses Ag-coated SiO2beads14,22; inacollection is driven by diffusion; inbcollection is driven by basic electrostatic precipitation through application of a bias voltage, whereIdreflects the rate of charge dissipation. (c) The concept of electrostatic precipitation is enhanced using an electrodynamic nanolens approach; a nanolens is formed using a patterned photoresist layer (PR) to funnel, concentrate, and spot the molecules at predetermined locations while preventing deposition on the positively charged resist. (d) The concept is further enhanced using electrically separated domains to receive different analytes at different times; domains are programmed by applying an external bias voltage. Inserts incandddepict scanning electron microscope and optical microscope images of the corresponding test structures and dimensions that were used. (c,d) Scale bar, 20 μm; (c, inset), 700 nm. Advanced collection, spotting and detection Figure 1 depicts the investigated design elements and test structures, which were evaluated to spot and collect airborne species on a nanostructured SERS gas sensor substrate. Figure 1a contrasts the state-of-the-art diffusion-based delivery concept with basic electrostatic precipitation, where an external bias and charged molecules are tested to increase the collection efficiency. Figure 1c adds an additional design element—a charged photoresist layer with a circular opening; the goal of this structure is to form an electrodynamic nanolens to funnel and concentrate the airborne species at a predetermined location on the nanostructured sensor surface. The use of a gas-phase nanolens focusing effect has been reported recently in the context of inorganic nanoparticles [23] , [24] , [25] , [26] that contained several 100,000 atoms, which contrasts with the small molecules tested here that contain less than 20 atoms. The general idea of a nanolens is to use a charged resist, which influences the trajectory of charged material. The resist serves as insulation and blocks charge dissipation. The opening to the conductor provides the only location where a charged material flux can be established under steady-state conditions. Figure 1d depicts an additional modification to achieve programmability of more than one analyte. The approach uses electrically separated metallic domains (yellow cap layers) underneath the nanolens array. Figure 1: Advanced localized collection and spotting of airborne species for gas sensor applications. ( a,b ) A nanostructured substrate commonly used in SERS called AgFON, which uses Ag-coated SiO 2 beads [14] , [22] ; in a collection is driven by diffusion; in b collection is driven by basic electrostatic precipitation through application of a bias voltage, where I d reflects the rate of charge dissipation. ( c ) The concept of electrostatic precipitation is enhanced using an electrodynamic nanolens approach; a nanolens is formed using a patterned photoresist layer (PR) to funnel, concentrate, and spot the molecules at predetermined locations while preventing deposition on the positively charged resist. ( d ) The concept is further enhanced using electrically separated domains to receive different analytes at different times; domains are programmed by applying an external bias voltage. Inserts in c and d depict scanning electron microscope and optical microscope images of the corresponding test structures and dimensions that were used. ( c , d ) Scale bar, 20 μm; ( c , inset), 700 nm. Full size image The fabrication of the depicted test structures is detailed in the methods section. In short, we used a Langmuir–Blodgett method [27] to apply a closely packed layer of silica spheres, 200 nm in diameter, over extended areas on the glass surface. Next, e-beam evaporation is used to coat the top with 20 and 180 nm of chromium and silver, respectively. This yields the SERS sensing surface commonly known in the literature as AgFON standard. The silver film provides a conductive layer. This conductive layer allows for the application of an external bias voltage, which is used to evaluate if a field driven approach can increase the collection efficiency of charge molecules when compared with prior concepts [14] , [15] , where the rate of absorption was driven by diffusion and the substrate was left floating. Prior methods were able to detect BTs at a concentration of 6 p.p.m. in 1 s. The second modification ( Fig. 1c ) adds the depicted 500-nm thick spin-coated photoresist layer whereby a 1 μm in diameter and 3 μm pitched hole pattern is defined by photolithography. The final SERS gas sensor substrate ( Fig. 1d ) is composed of two silver domains instead of one. The two domains are separated using a 50-μm wide region of uncoated silica spheres, which was masked by placing a capillary onto the surface prior metallization. All other parameters were left the same. The deposition on the individual domains is controlled using external bias voltages in the range of −50 to −200 V, whereby the electrometers records the deposition current in the range of 1–5 nA. The flux is recorded using electrometers (Keithley 6517A) marked with the letter ‘A’. Domains are turned ON and OFF sequentially for selected periods of time (10 s to 1 min) to collect molecular ions including BT + and 4-FBT + on domain 1 and 2, respectively. We choose these two molecules as they have a well-characterized and known Raman scattering signal [14] , [28] . The process is, however, not limited to these types of molecules or molecular weights. Results for anti-mouse IgG proteins (Sigma-Aldrich, F-0257) will be presented as well. 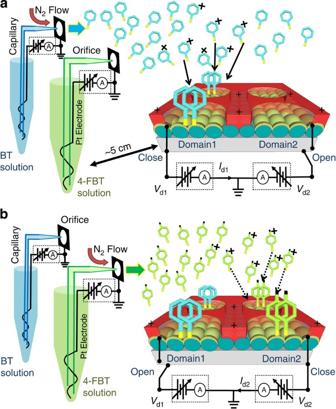Figure 2: Electrospray testing environment depicting electrospray ionization to produce a flux of neutral and charged analytes. (a) BT ions shown in light blue are selected to deposit on domain 1 in step 1. (b) 4-FBT ions shown in light green are selected to deposit on domain 2 in step 2. Circular 1 μm in diameter openings in the positively charged photoresist layer (red) act as a nanolens array, which concentrate the two analytes in predetermined sensing spots. The+sign on the red layer represents primary ionized carrier gas molecules. Switches marked as ‘open’ and ‘close’ are used to attract the analyte to the respective domains. Electrospray testing environment Figure 2 depicts the details of the testing environment where the analytes are evaporated and charged using an electrospray ionization standard and where programmable analyte collection is achieved using biased domain electrodes. Electrospray ionization is chosen as it provides a controlled environment to produce airborne analytes of almost any type and concentration. Electrospray ionization systems are used in mass spectroscopy in the fields of chemical-warfare agent detection [29] and proteomics [30] . They require exceptionally small amounts of diluted analytes. For example at a common flow rate, only 50 nl is drawn through the capillary per minute. For a review, we refer to Cloupeau and Prunet-Foch [31] and Ganan-Calvo et al. [32] . In brief, we constructed a system based on a commercially available electrospray ionization system (TSI Inc., Model 3480). It consists of a high-voltage source, pressure regulator, pressure chamber, capillary and electrospray chamber. The pressure chambers house a centrifuge vial, a high-voltage platinum electrode, and a fused silica capillary, which carries the solution out into the electrospray chamber using 1.25 atm pressure. A positive electrospray voltage is increased until the extruded liquid (50 nl per min) forms a cone shape, known as cone-jet mode [33] , which leads to rapid evaporation in close proximity to the orifice and an aerosol containing charged molecules (light green for 4-FBT, and light blue for BT). Figure 2: Electrospray testing environment depicting electrospray ionization to produce a flux of neutral and charged analytes. ( a ) BT ions shown in light blue are selected to deposit on domain 1 in step 1. ( b ) 4-FBT ions shown in light green are selected to deposit on domain 2 in step 2. Circular 1 μm in diameter openings in the positively charged photoresist layer (red) act as a nanolens array, which concentrate the two analytes in predetermined sensing spots. The+sign on the red layer represents primary ionized carrier gas molecules. Switches marked as ‘open’ and ‘close’ are used to attract the analyte to the respective domains. Full size image Figure 2a depicts the first analyte collection sequence where BT ions (BT + ) are collected on domain 1 which is turned ON by applying a negative voltage V d =−100 V to the domain electrode. Domain 2 is switched into a floating state, whereby the domain electrode is disconnected to prevent dissipation of charge, which in turn blocks the collection on domain 2. The following conditions were used to prepare the depicted ionized aerosol containing charged BTs. The starting point is a BT solution (liquid density=1.073 g/ml, molecular weight=110 g mol −1 ), which is diluted in a 1:1 volume ratio with ethanol; second, the solution is sprayed at a rate of 50 nl/min, which translates to 2.43 × 10 −7 N A BT molecules per minute, where N A is Avogadro’s constant; third, it is mixed with 1 liter per minute nitrogen carrier gas at 1.25 atm by adding 4.1 × 10 −2 N A nitrogen molecules per minute to the mixture; at this stage the analyte is diluted down to 5.9 p.p.m. In positive ion mode, the process produces positively charged molecules in addition to neutral molecules [34] . Of importance are BT ions (C 6 H 5 SH 2 + ), 4-FBT (C 6 H 4 FSH 2 + ), solvent ions (C 2 H 5 OH 2 + ) and nitrogen ions (N 2 + ). Figure 2b illustrates a second analyte collection sequence where 4-FBT + is collected on domain 2 and where domain 1 is left floating. The preparation approach for 4-fluorothiophenol (4-FBT) followed the same procedure as described before in the case of BT. The illustration in Fig. 2 under-represents the amount of neutral species for clarity. However, it is important to mention that most gas molecules are neutral and that the fraction of charged material is small. For example, a typical electrospray current is 100 nA, which is measured using the ampere metre marked with the letter ‘A’, which is connected to the platinum electrode that is immersed in the vial; 100 nA electrospray current translates into an ion current flux of 6.23 × 10 −11 N A elementary charges per minute. This ion flux is three orders of magnitudes smaller than the previously calculated 2.43 × 10 −7 N A BT molecules and nine orders of magnitudes smaller than 4.1 × 10 −2 N A nitrogen gas molecules contained in 1 l per min carrier gas. In other words, the gas mixture is composed of both charged (<1.5 p.p.b.) and neutral BT (<5.9 p.p.m.) molecules. The gas mixture exits the enclosed system through a 0.5 mm in diameter orifice and expands until it reaches the substrate, which is placed 5 cm away. The p.p.b. and p.p.m. estimates are upper limits and the actual concentration of charged and neutral molecules is smaller due to downstream mixture and charge exchange processes, which will be discussed further in the discussion section. 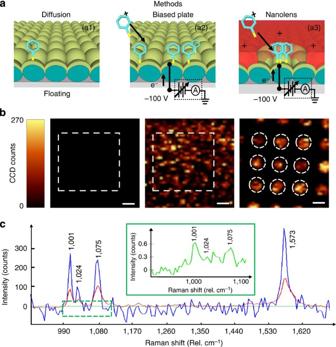Figure 3: Schematics and experimental results comparing different analyte collection concepts. Diffusion (LEFT), a biased plate (CENTRE), and a nanolens-based collection concept (RIGHT) all use a constant 30 s long exposure to a gas mixture containing both charged and neutral BTs. The biasing conditions depicted inalead tob, the recorded scanning confocal Raman intensity map of the characteristic Raman peak at 1,075 cm−1, and (c), corresponding spectra where the signal intensity for the biased substrates improves by a factor of 615. (b) Scale bar, 1 μm. Collection based on different mechanisms Figure 3 compares the recorded SERS signals using the floating, biased plate and biased nanolens collection approach after the test substrates were exposed for 30 s. The gas mixture exiting the electrospray system containing both charged (<1.5 p.p.b.) and neutral BT (<5.9 p.p.m.) molecules in nitrogen. All SERS spectra in Fig. 3c were recorded under identical exposure and recording conditions, which is important as this allows a relative comparison of the signal intensity for a sensor system with and without charge directed collection. For a standard SERS substrate, hotspots are randomly located on the surface ( Fig. 3b ) and it is hard to point out where the molecule is. The nanolens-based collection approach eliminates this uncertainty as molecules are collected at predetermined points ( Fig. 3c ). This helps in the data collection. In the particular case, all SERS spectra were recorded as an average over the indicated white dashed areas; no voltage is applied during the recording of the SERS data. The spectrum for the unbiased case shows a weak signal and the detection of the uncharged BT is difficult at 6 p.p.m. in our system; the characteristic peak at 1,075 cm −1 is recorded with 0.4 counts per unit area (inset of Fig. 3c ), which means very few BT molecules are collected on this substrate. The signal increases to 103 counts per unit area for the biased AgFON substrate and 246 counts per unit area for the biased AgFON substrate with integrated nanolens array, which represents a factor of 615 comparing the biased nanolens array with the unbiased AgFON standard. We repeated this experiment five times using separate substrates. The nanolens-based collection region produced the highest counts in each case; the intensity factor varied by 6% standard deviation (STD) between the experiments. The recorded increase of 615 is even more impressive if one considers that it is caused by 3,900 times fewer charged analyte molecules (1.5 p.p.b.) than neutral ones (5.9 p.p.m.). In other words, trace amounts of charged molecules at a concentration of 1.5 p.p.b. (parts per billion) lead to 246 counts per unit area, while 5.9 p.p.m. (parts per million) of neutral particles contribute to 0.4 counts, which means that the capture efficiencies of charged molecules is 2.4 × 10 6 times larger than neutral ones. The six orders of magnitude-higher capture efficiencies of charged molecules when compared with neutral one is an important metric, as it provides a route to higher sensitivity in any gas sensor application that presently uses diffusion as a mechanism of transport. Adding additional system components to charge the analyte to assist collection should yield similar gains. Figure 3: Schematics and experimental results comparing different analyte collection concepts. Diffusion (LEFT), a biased plate (CENTRE), and a nanolens-based collection concept (RIGHT) all use a constant 30 s long exposure to a gas mixture containing both charged and neutral BTs. The biasing conditions depicted in a lead to b , the recorded scanning confocal Raman intensity map of the characteristic Raman peak at 1,075 cm −1 , and ( c ), corresponding spectra where the signal intensity for the biased substrates improves by a factor of 615. ( b ) Scale bar, 1 μm. 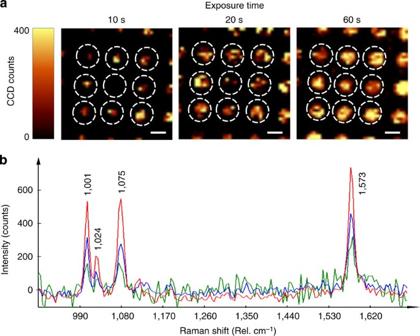Figure 4: SERS results for testing different collection times. SERS images (a) and spectra (b) for the localized nanolens enabled collection approach testing different collection times: 10 s (Left, green line), 20 s (Centre, blue line), and 60 s (Right, red line). (a) Scale bar, 1 μm. Full size image Localized nanolens enabled collection approach Figure 4a depict the Raman microscopy intensity map at 1,075 cm −1 Raman shift and spectra for the nanolens enabled collection approach as a function of collection time. The nanolens approach supports a more automated image processing that enables the elimination of the searching and hand picking of hotspots, which is a common practice in SERS-related measurements. Instead, we used a standard array of detection windows outlined with the dashed lines and averaging over these areas to record the spectra. The characteristic peaks at 1,001 cm −1 , 1,075 cm −1 and 1,573 cm −1 begin to emerge after a 10-s long exposure to charged BTs. For short periods of time, the signal increases roughly linear with exposure time and begins to level off after 60 s. For example, counts at the 1,001 cm −1 Raman shift are 170 (1 × ), 320 (1.9 × ), 540 (3.2 × ) for 10 s, 20 s, 60 s, respectively. This nonlinear behaviour and saturation for prolonged capture times can be explained by excessive packing of molecules, which are not as tightly coupled to the plasmonic surface [35] . For the same reason the signal-to-noise-ratio increases at first with exposure time before it levels off. Figure 4: SERS results for testing different collection times. SERS images ( a ) and spectra ( b ) for the localized nanolens enabled collection approach testing different collection times: 10 s (Left, green line), 20 s (Centre, blue line), and 60 s (Right, red line). ( a ) Scale bar, 1 μm. 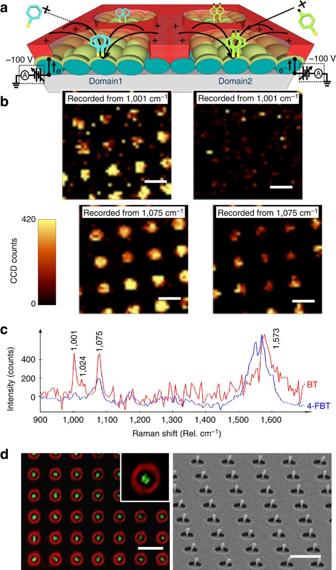Figure 5: Schematics and experiment results to spot and detect different molecules on a single substrate using programmable domain electrodes. (a) Schematic details the collection and SERS-based detection of BTs on the left and 4-FBT on the right. (b) Associated confocal Raman microscope intensity maps at wavenumbers 1,001 cm−1and 1,075 cm−1next to the (c) corresponding SERS spectra. (d) The fluorescent microscopy image shows the green fluorescence of large macromolecular anti-mouse IgG proteins, which are funneled into the photoresist hole pattern. (b) Scale bar, 1 μm; (d) 3 μm. Full size image Spot and detect different molecules on a single substrate Figure 5 illustrates experimental results where programmable domain electrodes are used to spot different molecules with different molecular weights, specifically BT (110.18 Da), 4-FBT (128.17 Da) and anti-mouse IgG (~150 kDa). The small molecules displayed characteristic Raman peaks that enable the recognition in the anticipated domains. As an example, domain 1 shows the presence of a peak at 1,001 cm −1 , which is known to be a dominant peak for the BT, which is not the case in 4-FBT in domain 2. Both molecules share a peak at 1,075 cm −1 , which represents a stretching mode of the aromatic ring. We would like to note that the intensity of the SERS signal depends on both the analyte amount and the localized plasmonic resonance. Plasmon resonances will only occur in the Ag layer and not on the photoresist surface. In other words, the absence of a SERS signal on the photoresist surface is not sufficient to conclude that there are no molecules on the photoresist. The previously presented increases in signal counts by a factor of 615 ( Fig. 3 ) comparing the biased nanolens array with an unbiased surface can, however, only be explained by an increased localized collection process. To further validate that material is only collected in the opening, we decided to use a fluorescence-based detection scheme and a much larger molecule in hope to image the location [36] using fluorescence microscopy. Specifically we tested anti-mouse IgG that is tagged with conventional fluorescence markers (fluorescein isothiocyanate, green). Figure 5d depicts the results. The fluorescence-based detection scheme decouples the detection mechanism from the plasmon resonant Ag layer. The intensity of the green fluorescence on the Ag surface and the absence of fluorescence on the photoresist surface can now be used as a measure of the selectivity with which the localized analyte delivery takes place. No detectable quantities of the IgG molecules are found on the photoresist and collection is observed only in the centre of the opening. Moreover, because IgG is three orders of magnitudes larger than the thiol molecules in this study, it was possible to resolve the location of physical analyte collection by scanning electron microscope. The molecules are confined to a 200 nm in diameter region, which is smaller than the 1 μm in diameter opening. Figure 5: Schematics and experiment results to spot and detect different molecules on a single substrate using programmable domain electrodes. ( a ) Schematic details the collection and SERS-based detection of BTs on the left and 4-FBT on the right. ( b ) Associated confocal Raman microscope intensity maps at wavenumbers 1,001 cm −1 and 1,075 cm −1 next to the ( c ) corresponding SERS spectra. ( d ) The fluorescent microscopy image shows the green fluorescence of large macromolecular anti-mouse IgG proteins, which are funneled into the photoresist hole pattern. ( b ) Scale bar, 1 μm; ( d ) 3 μm. Full size image The guided nanolens collection process and the results in Fig. 5d lead to the question of how the required fringing field is established and why continued deposition is only observed in the opening to the conductor. Our current hypothesis and understanding is that the deposition process is a self-equilibrating electrodynamic process whereby the electric field distribution evolves over time. In the initial stage of the experiment, ions respond to the external bias voltage that is applied to the domain electrodes. The smallest ions N 2 + have the highest mobility and arrive first at the sample surface. This transient response results in a sheath of space charge on the sample surface depicted as ’+’ on the red coloured photoresist layer within the illustrations, which alters the potential distribution. The potential distribution equilibrates and leads to a potential funnel where the analyte deposits in the centre of the opening. Steady-state charge dissipation can only occur in the opening and leads to a measurable flux of positive gas ions that includes the targeted molecules under a negative substrate bias, which is directly recorded using the electrometers (Keithley 6517A). An open discussion point relates to the ultimate sensitivity that may be achieved. The relative sensitivity increase in the case of the SERS sensor was 615 comparing the biased nanolens array with the unbiased AgFON standard, whereby the signal was caused by 3,900 times fewer charged analyte molecules than neutral ones. This yielded the 2.4 × 10 6 times larger capture efficiency for the charged molecules when compared with the neutral ones. This value has not be optimized and is based on the 1 μm in diameter and 3 μm pitched hole pattern shown in Fig. 1 ; higher values can be anticipated but would require optimization of the opening size, pitch, domain size and domain potential. For example a smaller pitch and higher potential should allow further increases. A corona charging method could also be employed to increase the charge ratio. Another discussion point relates to the actual concentration of the charged and neutral molecules at the sensor surface. The gas mixture that exits the enclosed electrospray system through the orifice plate contains roughly 5.9 p.p.m. (parts per million) neutral and 1.5 p.p.b. (parts per billion) charged analyte molecules, which was previously discussed in the paragraph describing Fig. 2 . However, additional dilution with the surrounding atmosphere will take place before the analyte reaches the substrate, which is placed 5 cm away in an otherwise open environment. The resulting additional dilution ratio can be calculated using a steady-state Gaussian plume model [37] , [38] where the downstream concentration as a function of distance depends upon the diameter of the orifice plate (0.5 mm) and cone shape where half-angle of the cone is ~9° (ref. 39 ) in our case yielding a cone diameter of 15.84 mm at the substrate location. Following the procedure published by Wein et al. [38] an additional analyte dilution factor of 1,003 will take place due to downstream mixing, which leads to ~1.49 p.p.t. (parts per trillion) charged analyte molecules and 5.88 p.p.b. (parts per billion) neutral analyte molecules at the sensor location. This is highly sensitive in absolute terms, which needs to be verified in further studies before this claim should be made. As a result, we used the upstream concentration at the orifice plate with 1.5 p.p.b. charged analyte molecules and 5.9 p.p.m. neutral ones to provide a conservative measure and a relative comparison. The overall conclusion remains as the recorded increase of 615 is caused by ‘at least’ 3,900 times fewer charged analyte molecules than neutral ones leading to an increased capture efficiencies of ‘at least’ 2.4 × 10 6 . The words ‘at least’ account for the fact that additional dilution takes place and that further gains through optimization of the opening size, pitch, domain size and domain potential can be anticipated. The reported process can also be used as a programmable selected area deposition or surface treatment method with molecular ions. The sequence and amount can be mixed and matched with a lateral resolution that is several orders of magnitudes higher than what is possible using existing methods that are based on mechanical shutters or high-precision contact-printing robots. The ability to fabricate hybrid molecular arrays with control over material sequence, composition and lateral distribution on a single substrate within a single process could potentially be used in other applications, which include, proteomics and cell research, pharmaceutical screening processes, panel immunoassays and molecular electronics [20] , [21] , [40] . In conclusion, various nanostructured sensors currently aim to claim single molecular detection by a reduction of the active sensor size. An equally important challenge, however, can be found in the question ‘whether the analyte will ever find the nanometre sized surface’. The smaller the sensor, the less likely the probability for a molecule to attach to the sensor surface considering a diffusion-based detection system. The reduction in the size of the active sensor will ultimately require research on methods that enable localized delivery. The reported electrodynamic collection concept is a first step in this direction. Materials All chemicals were reagent grade and used as received. Surfactant-free, silica nanosphere suspensions (200 nm, 4 wt %) were acquired from Bangs Laboratories, Inc. BT and 4-FBT were purchased from Sigma-Aldrich (Milwaukee, WI). NH4OH, H2O2, and H2SO4 were purchased from Fisher Scientific (Fairlawn, VA). AgFON fabrication Glass slides (75 mm long, 50 mm wide, 1 mm thick) were first pretreated in piranha etch at 120 °C for 30 min, and then in 5:1:1 ratio of H 2 O:NH 4 OH:H 2 O 2 for 30 min to make the surface hydrophilic. The 200 nm monodisperse silica nanosphere suspension (4% silica spheres by weight in water) was further diluted in ethanol (1:1 volume ratio). The ethanol served as a spreading agent, which we found to help in the next step. The 2 μl suspension was carefully dropped onto the water surface which yields a surface layer of silica beads. The Langmuir–Blodgett method was used to compact the beads and to transfer the beads to the target slide. After drying the surface for 30 min, the AgFON standard substrate was completed through e-beam evaporation of 20 nm chromium and 180 nm silver to form the plasmonic cap layer. The silver thickness and deposition rate were measured by a 6 MHz quartz crystal microbalance from INFICON (East Syracuse, NY). Nanolens array The nanolens array is composed of a patterned photoresist layer. Photoresist (Microposit 1805, Shipley) was spin coated at 3,000 rpm for 40 s on an AgFON substrate. After soft-bake at 105 °C for 1 min, the substrate was photolithographically patterned with the 96 mJ cm −2 ultraviolet light and developed in a developer (Microposit 351:H 2 O=1:5) for 25 s. A 15 s oxygen plasma cleaning step was used to remove any residues. The substrates were thoroughly rinsed with deionized water and blown dry with high purity nitrogen (99.998%) before they were used. The electrodynamic nanolens pattern was composed of 1 μm diameter holes on a 3-μm pitch. In the initial stage, the photoresist becomes charged and equilibrates as a consequence of the ionic deposition process. The charged resist deflects and guides charged ions into the opening. Programmable nanolens array The programmable nanolens array used the same substrate and same photoresist film as described before. The only difference is that the Cr/Ag film is defined into separated domains to allow for the application of separate bias voltages to control the deposition in each domain. The domains are separated by a 50-μm wide region, which was not coated with silver. The region was masked using a 50 μm in diameter capillary during the e-beam evaporation of 20 nm chromium and 180 nm silver to form electrically separated plasmonic cap layers. Characterization A scanning electron microscope (JEOL 6500) was used to examine the surface morphology of AgFON substrates and measure the size. SERS spectra and two-dimensional confocal microscopy scanning images were acquired using a confocal Raman microscope system (Witec Alpha 300R) equipped with a 100 × objective lens (Nikon 100 × , 0.90 NA in air). A fibre-optic interfaced 514 nm argon ion laser was used as the laser source. The laser power was maintained constant and set to ~2 mW within one experimental set of measurements. The lateral imaging resolution of the confocal system considering the wavelength, and numerical aperture of the system is ~300 nm. The scattered light was analysed using a 600 mm −1 spectrometer grating with a spectral resolution of about 3 cm −1 . The collection time for each raster spot constant was 1 s. SERS spectra were collected from multiple spots across the substrate and from multiple substrates. The reflectance absorption spectrum was analysed using an optical fibre VIS-NIR spectrophotometer (Ocean Optics, USB4000 VIS-NIR spectrometer, QR400-7-UV–vis reflection probe). The reflectance absorption spectrum of AgFON was collected and used for the chosen wavelength (514.5 nm). How to cite this article: Lin, E.C. et al. Effective localized collection and identification of airborne species through electrodynamic precipitation and SERS-based detection. Nat. Commun. 4:1636 doi: 10.1038/ncomms2590 (2013).